Stretchable heterogeneous composites with extreme mechanical gradients Heterogeneous composite materials with variable local stiffness are widespread in nature, but are far less explored in engineering structural applications. The development of heterogeneous synthetic composites with locally tuned elastic properties would allow us to extend the lifetime of functional devices with mechanically incompatible interfaces, and to create new enabling materials for applications ranging from flexible electronics to regenerative medicine. Here we show that heterogeneous composites with local elastic moduli tunable over five orders of magnitude can be prepared through the site-specific reinforcement of an entangled elastomeric matrix at progressively larger length scales. Using such a hierarchical reinforcement approach, we designed and produced composites exhibiting regions with extreme soft-to-hard transitions, while still being reversibly stretchable up to 350%. The implementation of the proposed methodology in a mechanically challenging application is illustrated here with the development of locally stiff and globally stretchable substrates for flexible electronics. Integration of different synthetic materials, such as polymers, metals and ceramics, into functional devices often results in mismatches in mechanical and thermal properties that favour premature failure of the solid interfaces due to stress localization. Examples of functional devices whose durability is impaired by premature interfacial failure are numerous and range from biomedical implants in orthopaedics [1] to metal-composite joints in automotive and aerospace applications [2] , [3] to inorganic functional devices in high-performance flexible electronics [4] . In some applications, this issue can be circumvented by developing functionally graded heterogeneous materials whose through-thickness chemical composition is gradually changed to reduce mismatches in the elastic and thermal properties of the homogeneous materials to be integrated. However, this approach has been limited to purely inorganic systems whose elastic moduli lie within the same order of magnitude, as is the case for example of ceramic thermal barrier coatings deposited on metals [5] , [6] . Constructing heterogeneous composite materials with locally tuned mechanical properties in all three dimensions is a recurring strategy in nature to achieve unusual mechanical properties and to couple surfaces with very different elastic moduli [7] , [8] , [9] , [10] , [11] , [12] , [13] , [14] . For instance, the biological tissue that connects tendons to bone exhibits locally tuned elastic moduli that can vary by as much as two orders of magnitude to match the stiff surface of bone with the soft tendon [15] , [16] , [17] . This is achieved by changing the local concentration of hydroxyapatite reinforcing particles embedded within hierarchically structured collagen fibres [15] . Similarly, the teeth of many vertebrates and invertebrates exhibit a three-dimensional (3D) bilayer structure that combines a remarkable surface hardness to withstand mastication loads with a high toughness in the inner layer to resist crack propagation. Such properties are achieved by tailoring the concentration and orientation of reinforcing mineral particles across the material [12] , [18] . Although a multitude of other heterogeneous natural composites with locally tuned elastic moduli exist [9] , [18] , [19] , [20] , the examples above well illustrate the ability of biological materials to deliberately control its mechanical properties by using an entangled continuous polymer matrix reinforced to different extents with a limited choice of inorganic reinforcing elements [21] , [22] . Such an interpenetrating polymer matrix is believed to be key in ensuring efficient stress transfer and in avoiding local failure between regions of different elastic moduli. Despite the improved mechanical and thermal interfacial coupling offered by artificial functionally graded heterogeneous materials, the 3D nature and the unique local control of structure and properties observed in heterogeneous biological composites have not yet been achieved in synthetic systems. Obtaining such level of 3D control in artificial heterogeneous composites would allow us to not only extend the lifetime of existing functional devices prone to interfacial failure but also to develop new materials for mechanically challenging demands. These include for example dental restorations for prosthetic dentistry that more closely resemble the mechanical properties of natural tooth [23] , elastomeric substrates for flexible electronics that are bendable and stretchable but yet locally stiff [24] , [25] , [26] , [27] , [28] , [29] and synthetic bio-scaffolds for the replacement of intervertebral discs [30] and for the regeneration of graded tendon/ligament-to-bone insertions [31] , [32] , [33] . In addition to addressing such mechanical challenges, the deliberate local reinforcement of weak regions achievable with such heterogeneous composites also represents an economical and environmental-friendly approach to attain the required mechanical performance while minimizing the use of limited and costly resources. Here we show that heterogeneous manufactured composites exhibiting elastic moduli spanning over several orders of magnitude can be obtained by tuning the local reinforcement of an entangled continuous polymer matrix using reinforcing elements at multiple hierarchical levels. To illustrate the unusual sets of properties that can be achieved with this approach, we create 3D polymer-based composites whose local elastic modulus on the surface can approach that of the hardest biological materials such as bone and tooth enamel, whereas still being reversibly stretchable up to 350% strain on a global scale without failure. Hierarchical composites with extreme mechanical gradients Composites with different elastic moduli were created by hierarchically reinforcing a polyurethane (PU) soft matrix with (1) PU hard segment domains, (2) inorganic nanoplatelets and (3) inorganic microplatelets at progressively larger length scales ( Fig. 1a ). Reinforcement of the soft PU matrix with PU hard segments is accomplished by increasing the relative fraction of hard-to-soft segments (HS:SS) during PU synthesis ( Fig. 1a ). Further stiffening of PU matrices is achieved through the selective reinforcement of the PU hard domains with laponite nanoplatelets, following the procedure developed by Liff et al . [34] , [35] . Alumina microplatelets are finally used to reinforce the laponite-containing PU matrix at the next hierarchical level. Following this procedure, we produce individual PU films with elastic moduli that can be tuned between 4 MPa and 7 GPa [34] . In Fig. 1a , the individual PU compositions are indicated by the letter M followed by their elastic moduli in MPa. 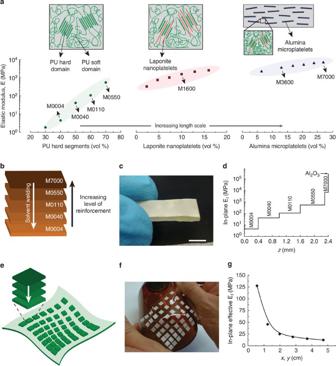Figure 1: Hierarchical heterogeneous composites with locally tuned elastic properties. (a) Elastic modulus of PU-based composites reinforced with different volume fractions of hard segments (left), laponite nanoplatelets (centre) and alumina microplatelets (right) at increasing hierarchical levels. Arrows indicate the compositions of reinforced PUs used in this study, which are identified by the letter M followed by their elastic moduli in MPa units. (b–d) Heterogeneous composite with extreme elastic gradient in the out-of-plane direction (d) prepared through solvent welding of individual layers with different reinforcement levels and atomic layer deposition of a 100 nm-thick alumina layer (b). The solid black line indindicates the in-plane elastic modulus as a function of the sample heightz. (e–g) 3D heterogeneous composite with tunable elastic moduli in the out-of-plane and in the in-plane directions made by welding modular patches onto an elastomeric PU film (e). Graph (g) shows the effective elastic modulus of the 3D composite in the in-plane direction. (c) Scale bar, 5 mm. Figure 1: Hierarchical heterogeneous composites with locally tuned elastic properties. ( a ) Elastic modulus of PU-based composites reinforced with different volume fractions of hard segments (left), laponite nanoplatelets (centre) and alumina microplatelets (right) at increasing hierarchical levels. Arrows indicate the compositions of reinforced PUs used in this study, which are identified by the letter M followed by their elastic moduli in MPa units. ( b – d ) Heterogeneous composite with extreme elastic gradient in the out-of-plane direction ( d ) prepared through solvent welding of individual layers with different reinforcement levels and atomic layer deposition of a 100 nm-thick alumina layer ( b ). The solid black line in d indicates the in-plane elastic modulus as a function of the sample height z . ( e – g ) 3D heterogeneous composite with tunable elastic moduli in the out-of-plane and in the in-plane directions made by welding modular patches onto an elastomeric PU film ( e ). Graph ( g ) shows the effective elastic modulus of the 3D composite in the in-plane direction. ( c ) Scale bar, 5 mm. Full size image Heterogeneous composites with deliberate local stiffness are prepared by solvent-welding individual films with different levels of reinforcements into one single component, as schematically illustrated in Fig. 1b . In the solvent-welding process, two film surfaces are first wetted by a good solvent and pressed together to allow for polymer entanglement, which is then preserved upon solvent evaporation. Such entanglement eliminates the interfaces between individual films, leading to heterogeneous composites with efficient stress transfer throughout the structure. The upper limit in elastic modulus achieved with the hierarchical polymer-based composite (7 GPa) can be further increased on the surface through the deposition of a 100 nm-thick layer of Al 2 O 3 via atomic layer deposition (150 °C per 160 min) [36] . Using this approach, we obtained 2 mm-thick heterogeneous composites with an out-of-plane gradient in elastic modulus spanning over five orders of magnitude ( Fig. 1c ). The resulting composite is locally stiffer than tooth enamel on one side ( E l ~10 2 GPa), whereas being softer than skin on the other ( E l ~1–5 MPa, see Fig. 1d ). The extreme span in stiffness achievable within a single material free of macroscopic interfaces is far greater than that of other artificial graded composites [32] and is comparable to that of highly graded biological materials [20] . This opens numerous possibilities for the design of synthetic heterogeneous composites with deliberate local mechanics. For instance, modular patches with any predefined E l -profile can be solvent-welded at different preselected locations on the surface of a polymer substrate to create 3D composites with tunable elastic modulus profiles in the in-plane and out-of-plane directions ( Fig. 1e ). In this example, not only the internal microstructure but also the shape of the composite is designed to effectively fulfil a mechanical function, alike the design strategy of many biological materials. The out-of-plane E l -profile is determined by the local concentration of reinforcing elements throughout the cross-section of each modular patch at the microscale. The in-plane E l -profile is controlled by the geometry and average elastic moduli of the patches and of the underlying substrate at the macroscale ( Fig. 1g and Supplementary Methods ). All these parameters can be varied independently and in a modular fashion, providing a wide design space for tailoring the local elastic moduli of the heterogeneous composite in both the in-plane and out-of-plane directions. Finite element analysis of composite architectures To further explore the unusual set of properties offered by 3D heterogeneous composites with tailored E l profiles, we investigated specific architectures that would combine high global stretchability with minimum local strains at specific surface sites. The response of 3D composites with deliberate E l profiles to stretching is first evaluated by simulating the local mechanical stresses and strains across representative patch–substrate modules using finite element analysis (FEA) ( Fig. 2 ). Each module consists of a prismatic patch with designed E l profile deposited onto a ribbon of stretchable substrate. Four different patch–substrate module designs were investigated: two with a constant E l across the patch, one with a graded E l profile, and one control module with patch and substrate of same elastic modulus. These different hypothetical arrangements are shown in Fig. 2a and referred to throughout the text using the letter S followed by the elastic modulus of the patch (except for the graded patch, which is named S-Grad). 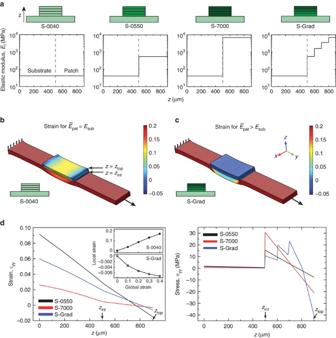Figure 2: FEA of the local mechanics of representative patch–substrate modules with tunable elastic properties. (a) Elastic modulus profiles of the investigated modules, which are identified by the letter S followed by the assumed elastic moduli in MPa units. (b,c) Distribution of strainsεyyfor the architectures S-0040 and S-Grad after applying a longitudinal global strain (εg) of 25% in they-direction. (d)εyy(left) andσyy(right) profiles across the height of different patch–substrate architectures (εg=25%). The inset shows the variation of the local strain (εyy) at the centre of the top surface of the patch as a function of the global strain (εg) applied to the substrate for the S-0040 and S-Grad modules. Figure 2: FEA of the local mechanics of representative patch–substrate modules with tunable elastic properties. ( a ) Elastic modulus profiles of the investigated modules, which are identified by the letter S followed by the assumed elastic moduli in MPa units. ( b , c ) Distribution of strains ε yy for the architectures S-0040 and S-Grad after applying a longitudinal global strain ( ε g ) of 25% in the y -direction. ( d ) ε yy (left) and σ yy (right) profiles across the height of different patch–substrate architectures ( ε g =25%). The inset shows the variation of the local strain ( ε yy ) at the centre of the top surface of the patch as a function of the global strain ( ε g ) applied to the substrate for the S-0040 and S-Grad modules. Full size image FEA revealed that patches respond differently to the external tensile strain, depending on whether their average elastic moduli ( Ē pat ) are equal or higher than that of the underlying substrate ( E sub ). For Ē pat > E sub , patches undergo significant inward bending during tensile stretching of the representative modules. This effect generates compressive (negative) strains on the patch surface and tensile (positive) strains across the substrate, as shown in Fig. 2c . In contrast, the patch exhibiting the same elastic modulus as the substrate ( Ē pat = E sub , S-0040) experiences a combination of bending and stretching. This leads to curved surfaces at the edge of the patch and a stretched area with high tensile strains at its centre ( Fig. 2b and Supplementary Fig. S1 ). Among the patches with Ē pat > E sub , we observe that bending becomes less pronounced as the average stiffness of the patch increases (higher Ē pat ). The radius of curvature of the region that underwent bending was found to be 9.7, 17.2 and 63.2 mm for the specimens S-0550, S-Grad and S-7000, respectively. As a result, the stiffest patch (S-7000) offers the advantage of a lower compressive strain on the top surface and a lower tensile strain at the bottom of the underlying substrate ( Fig. 2d ). Because of its stiff top layer, the graded patch (S-Grad) experiences surface compressive strains nearly as low as that of the stiffest patch (S-7000). In addition to the strains at the surface, the elastic modulus profile of the patch also affects the mechanical stability and stretchability of the module, as local mismatches in E l may cause excessive stress concentrations within the structure and thus premature failure of the composite upon stretching. Analysis of the stress distribution throughout the cross-section of the simulated modules revealed the expected stress peaks at regions where the elastic modulus changes abruptly ( Fig. 2d ). Although the stress and strain indicated in Fig. 2d refer only to the normal values at the centre of the patch, similar trends were observed for the shear values at the edge of the simulated patches (see Supplementary Fig. S2 ). The less abrupt changes in local elastic modulus throughout the architectures S-0550 and S-Grad lead to lower tensile stress peaks and thus a presumably higher resistance against local delamination during stretching. Because of its graded architecture, the module S-Grad better distributes the stress along the height of the patch, which contrasts to the sharp stress peak observed at the bottom of the stiffest homogeneous patch (S-7000, z = z int ). Overall, the FEA indicate that the graded architecture is the most suited to minimize the strain on the patch surface, whereas preventing premature failure of the stretched composites through reduced mechanical mismatches throughout the structure. Combining ultra-stretchability with local surface stiffness To experimentally investigate the surface strains and the failure resistance of composites exhibiting architecture similar to the S-Grad design, we fabricated graded modules using the hierarchical reinforcement approach described above (E-Grad, Fig. 3 ). A highly stretchable, fully recoverable elastomeric substrate ( Fig. 3a ) was produced by performing a two-step polymerization reaction of a 50:50 weight ratio mixture of hard and soft monomers in N,N -dimethylformamide (DMF), followed by casting in a silicone rubber mould (see details in the Supplementary Methods ). Mechanically graded patches were formed by solvent welding and hot pressing individual layers with progressively higher elastic modulus using DMF as solvent. The elastic modulus was tuned to gradually increase from the bottom to the top of the patch by changing the type and concentration of reinforcing elements, as depicted in Fig. 3b . A freeze-fractured cross-section of the resulting graded sample exhibits a very smooth surface across the platelet-free PU layers and no detectable interface between the platelet-reinforced layers ( Fig. 3c ). This suggests that the macromolecules of the different original layers are effectively entangled and that a graded structure containing an interpenetrating polymer matrix was successfully created. 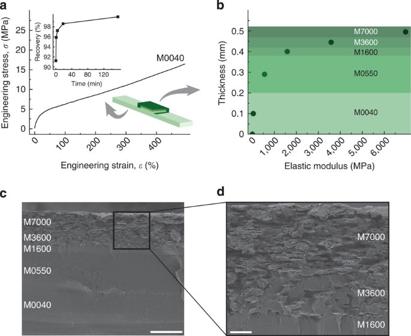Figure 3: Mechanics and microstructure of synthetic heterogeneous composites with graded patch architecture. Materials are identified by the letter M followed by their elastic moduli in MPa units. (a) Stress–strain behaviour for the elastomeric PU containing 50% of hard segments used as underlying substrate (strain rate: 2.5 mm min−1). The inset shows the full recoverability of the elastomer after a strain of 80% is released at room temperature. (b) In-plane elastic modulus profile across the height (z) of the graded patch. (c,d) SEM images of the graded patch highlighting the absence of macroscopic interfaces after solvent welding. Scale bar, 100 μm (c) and 20 μm (d). Figure 3: Mechanics and microstructure of synthetic heterogeneous composites with graded patch architecture. Materials are identified by the letter M followed by their elastic moduli in MPa units. ( a ) Stress–strain behaviour for the elastomeric PU containing 50% of hard segments used as underlying substrate (strain rate: 2.5 mm min −1 ). The inset shows the full recoverability of the elastomer after a strain of 80% is released at room temperature. ( b ) In-plane elastic modulus profile across the height ( z ) of the graded patch. ( c , d ) SEM images of the graded patch highlighting the absence of macroscopic interfaces after solvent welding. Scale bar, 100 μm ( c ) and 20 μm ( d ). Full size image The effectiveness of the entangled polymeric matrix and the elastic modulus gradient in increasing the composite failure resistance was investigated by performing tensile tests on graded (E-Grad) and non-graded (E-7000) experimental samples prepared as described above. Remarkably, substrates containing the graded patch could be stretched by as much as 350% without failure due to localized internal stresses ( Fig. 4a ). The high shear stresses developed at the interface between the substrate and the graded patch close to the patch edge (see Supplementary Fig. S2c ) lead to partial detachment of the substrate for global tensile strains >150% (see white arrow in Fig. 4b ). However, because of the lower stresses developed within the graded patch as compared with the non-graded stiff patch (S-Grad and S-7000 in Supplementary Fig. S2 ), this partial detachment is limited to the edge of the graded patch and does not lead to complete delamination of the patch–substrate interface ( Fig. 4b and Supplementary Fig. S3 ). Instead, failure of the patch–substrate module typically occurs through the rupture of the elastomeric substrate material close to the patch edge at global strains >350% without delamination ( Supplementary Fig. S4 ). This indicates that mechanical degradation in this system is controlled by the tensile strength of the substrate material rather than the strength of the patch–substrate interface, which allows us to take full advantage of the high stretchability of the elastomeric substrate. In contrast, composites exhibiting a homogeneous patch of the stiffest material (E-7000) delaminated completely at the interface between the patch and the substrate at strains between 150 and 200%. These results qualitatively agree with the FEA and can be explained by the lower stress concentration at the patch–substrate interface predicted for the graded composite ( Fig. 2d ). 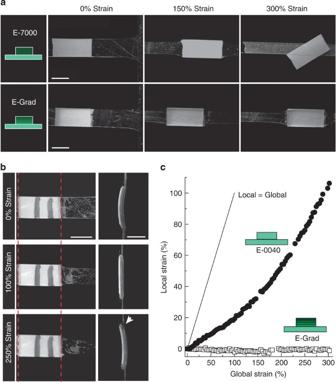Figure 4: Failure resistance and local surface strain of synthetic graded composites in comparison with non-graded controls. The experimental samples are identified by the letter E followed by the elastic modulus of the patches in MPa. (a) Resistance of the graded architecture against interfacial failure under stretching as opposed to the complete delamination observed for the non-graded sample containing the stiffest patch. (b) Front and lateral views of graded specimens (E-Grad) under increasing global tensile strains, highlighting the inward bending of the patch upon stretching. The white arrow indicates only partial detachment of the substrate at the edge of the graded patch. (c) Local strain <1% on the surface of graded patches for increasing global tensile strains, as opposed to the increasing local deformations observed for the control sample. (a,b) Scale bars, 2 mm. Figure 4: Failure resistance and local surface strain of synthetic graded composites in comparison with non-graded controls. The experimental samples are identified by the letter E followed by the elastic modulus of the patches in MPa. ( a ) Resistance of the graded architecture against interfacial failure under stretching as opposed to the complete delamination observed for the non-graded sample containing the stiffest patch. ( b ) Front and lateral views of graded specimens (E-Grad) under increasing global tensile strains, highlighting the inward bending of the patch upon stretching. The white arrow indicates only partial detachment of the substrate at the edge of the graded patch. ( c ) Local strain <1% on the surface of graded patches for increasing global tensile strains, as opposed to the increasing local deformations observed for the control sample. ( a , b ) Scale bars, 2 mm. Full size image Tensile mechanical tests were conducted to experimentally assess the local strain on the surface of graded (E-Grad) and non-graded (E-0040) patches as a function of increasing global deformations. The local strain was obtained by measuring the length of the patch on lateral images acquired by a travelling microscope during mechanical deformation ( Fig. 4b ). In line with the FEA predictions, local strains <1% were detected on the surface of the graded patch for global strains as high as 300%. Conversely, samples consisting of both patch and substrate made of the same PU (E-0040, Ē pat = E sub ) displayed the predicted steady increase in local tensile strain for increasing global strains ( Fig. 4c and inset of Fig. 2d ). The inward bending effect observed in the simulation of the graded composite was confirmed by lateral recording of the specimen during the tensile test ( Fig. 4b ). Interestingly, the as-prepared graded patch developed an outward curvature after solvent welding and hot pressing the individual composite layers. This initial outward bending presumably results from the higher shrinkage of the substrate and the softer bottom layers of the graded patch upon removal of the welding solvent and release of the load applied during hot pressing. Graded composites for stretchable electronics To demonstrate the potential of such 3D-graded composites in combining unusual functional properties, we deposited a 50-nm conductive gold layer on the top surface of the graded patch and measured its electrical response while stretching the underlying elastomeric substrate ( Fig. 5a ). Because of its small thickness and poor interfacial adhesion, the gold layer is expected to start deforming and to exhibit increasing electrical resistance at tensile strains of about 1% [27] ; thus, much earlier than its strain-at-rupture of 20–30% [27] , [37] . As the strain of 1% is comparable to the failure tensile strain of high-performance semiconductor and dielectric layers (for example indium–gallium–zinc oxide and aluminium oxide) [4] , the electrical response of the gold layer can be taken as a simple indicator of the effectiveness of the graded composites in protecting brittle electronic devices in stretchable electronic applications. The stretching experiments revealed that the 3D graded composite can be globally strained by as much as 200% without any detectable increase in the electrical resistance of the gold layer ( Fig. 5a ). This is in strong contrast with the sharp increase in resistance at ~1–2% strain obtained for a control sample consisting of a gold layer deposited directly on the elastomeric substrate. 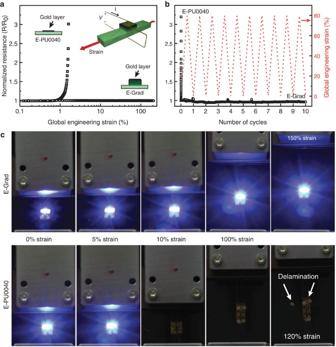Figure 5: Electrical responses of a conductive film and a functional electronic device subjected to steady or cyclic tensile strains. (a) Normalized electrical resistance of a thin gold layer deposited on the surface of a graded patch (E-Grad) or directly on the elastomeric substrate (E-PU0040) as a function of steadily increasing global strains. The inset schematically shows the setup used for the simultaneous electrical and mechanical measurements. (b) Normalized electrical resistance of the gold layer deposited on the same specimens shown inawhen subjecting the substrate to cyclic strains with a maximum amplitude of 80% (c) Steady stretching of patch–substrate modules containing a switched-on LED assembled on the patch surface. The diode assembled on the graded patch (E-Grad) remains functional up to global strains as high as 150%, whereas it fails and eventually delaminates before 10% strain if deposited directly on the elastomeric substrate (E-PU0040). Figure 5: Electrical responses of a conductive film and a functional electronic device subjected to steady or cyclic tensile strains. ( a ) Normalized electrical resistance of a thin gold layer deposited on the surface of a graded patch (E-Grad) or directly on the elastomeric substrate (E-PU0040) as a function of steadily increasing global strains. The inset schematically shows the setup used for the simultaneous electrical and mechanical measurements. ( b ) Normalized electrical resistance of the gold layer deposited on the same specimens shown in a when subjecting the substrate to cyclic strains with a maximum amplitude of 80% ( c ) Steady stretching of patch–substrate modules containing a switched-on LED assembled on the patch surface. The diode assembled on the graded patch (E-Grad) remains functional up to global strains as high as 150%, whereas it fails and eventually delaminates before 10% strain if deposited directly on the elastomeric substrate (E-PU0040). Full size image The protection of brittle electronic devices over prolonged periods of time requires substrates that are not only highly stretchable but that can also withstand extensive cyclic deformation. The resistance of the proposed 3D graded composites against cyclic strains was probed by following the electrical resistance of the conductive gold layer while subjecting the underlying elastomeric substrate to a cyclic triangular strain pattern with maximum engineering strain of 80%. In contrast to the sharp increase in resistivity observed in the first stretching cycle of a control sample, the 3D-graded composite was able to keep the gold layer fully conductive and with no detectable increase in electrical resistance after more than 10 full cycles ( Fig. 5b ). The ability of the 3D-graded architecture to protect brittle electronic devices was ultimately probed by assembling a light-emitting diode (LED) on the surface of a graded patch and testing its function while increasing tensile strains was applied to the substrate beneath. By using silver paste, the diode was electrically contacted to two sputtered gold layers connected to a 9V external battery and finally fixed in place with epoxy glue. Upon stretching of the whole construct, the switched-on LED deposited on the graded patch remained functional up to 150% global strain, as opposed to the impaired functionality and delamination observed for control diodes assembled directly onto the elastomeric substrate ( Fig. 5c ). Although elegant photolithographic approaches have been successful in locally increasing the elastic modulus of polydimethylsiloxane elastomers within the MPa range by a factor of 5 (refs 25 , 38 ), the 100-fold reduction in the local-to-global strain ratio enabled by the graded architecture outperforms previous attempts to obtain locally stiff islands that protect brittle inorganic layers from failure in stretchable electronics [25] , [26] , [27] , [28] , [29] . As the step at the patch edges might be undesired in flexible electronics, other geometries can be readily obtained using other approaches to assemble the PU compositions with different level of reinforcement, including hot-pressing, tape-casting, screen-printing and 3D rapid prototyping techniques. As an illustrative example, we produced a planar substrate with locally reinforced islands by simply hot-pressing graded patches into an elastomeric thick layer ( Supplementary Fig. S5 ). The step between the pressed patch and the elastomeric substrate is <15.2 μm, which enables sputtering of conductive metallic interconnectors between LEDs assembled onto adjacent islands ( Supplementary Figure S6 ). Using this flat configuration, in-plane gradients at the edge of the patch can potentially be also introduced using individual layers of different sizes to eliminate the stress concentration leading to partial detachment of the substrate at the patch edge ( Fig. 4b and Supplementary Fig. S3 ). In addition to the macroscopic LEDs shown in Fig. 5c , our recent demonstration that high-performance thin film transistors can be deposited and successfully operated on the surface of platelet-reinforced polymeric substrates [26] confirms the great potential of using such graded, hierarchical composites in stretchable electronics and other functional devices requiring extreme gradients in elastic modulus, including flexible solar cells, circuit boards, biological sensors and wearable electronic devices. The proposed methodology could be further improved by exploring approaches to increase the thickness and the smoothness of the purely inorganic layer deposited on the hard side of the reinforced composite. In summary, we show that tuning of the local reinforcement level of a thermoplastic elastomer in 3D can lead to polymer-based heterogeneous composites with unique set of mechanical properties within the same material, including for example millimetre-thick profiled sheets with an out-of-plane soft-to-hard transition spanning 2 decades in elastic modulus combined with a global in-plane stretchability >350%. Such properties are achieved by reinforcing the soft elastomeric polymer matrix with hard molecular domains, nanoplatelets and microplatelets at progressively higher hierarchical levels and at deliberate positions of the composite. Spatial control over the reinforcement level is possible by solvent welding individual layers with different concentrations of reinforcing elements. Our ability to create heterogeneous composites with locally tunable elastic modulus spanning over five orders of magnitude with a fully entangled polymer phase allows us to combine unusual functional properties that would not be achievable with homogeneous materials. In addition to the locally stiff and globally stretchable substrates demonstrated here, this method can potentially be explored to produce artificial biomaterials with extreme mechanical gradients for cartilage, tendon and ligament repair in regenerative medicine, durable dental restorations that more closely match the flaw-tolerant architecture of natural tooth, and tougher graded adhesives that would reduce catastrophic failure of current fiber-reinforced composites. The approach may also be exploited to create bioinspired heterogeneous architectures that mimic the structural features of biological materials, allowing for the investigation of biological structure–function relationships of interest for reverse biomimetics [39] . Materials All chemicals were purchased from Aldrich Co. and were of analytical grade, unless otherwise stated. DMF (dried over molecular sieves), 4,4′-methylenebis(cyclohexyl isocyanate) (H-MDI, 90%), 1,4-butanediol (BDO,≥99%); poly(tetrahydrofuran) (T1000, M w =1,000 g mol −1 ), glycerol ethoxylate (EG, M w =1,000 g mol −1 ) and dibutyltin dilaurate were used for the synthesis of PUs with different HS:SS ratios. Composites were prepared using a commercial thermoplastic PU (Elastollan C64D, BASF, Germany), DMF (ACS grade), polyvinylpyrrolidone (PVP, M w =40,000 g mol −1 ), alumina platelets with average diameter of 7.5 μm and thickness of 200 nm (Alusion, Antaria Limited, Australia) and laponite platelets with diameter of 25 nm and thickness of 1 nm (Laponite RD, ProChem, Switzerland). PU syntheses PU syntheses were carried out under nitrogen atmosphere in a three-neck round-bottom flask equipped with a reflux condenser. H-MDI and BDO were used as hard segments, T1000 as soft segment and EG as cross-linker. The HS:SS ratio was adjusted by changing the proportion between T1000 and BDO. First, the glassware was dried with a heating gun at 350 °C to remove any adsorbed water. Then, a prepolymer was prepared by loading the flask with H-MDI followed by the dropwise addition of a solution of T1000 and EG in DMF under magnetic stirring (600 r.p.m). The resulting mixture was kept at 80 °C for 3 h. After formation of the prepolymer, the temperature was reduced to 60 °C and a solution of BDO in DMF was added to the flask to proceed with the polymerization reaction for a time period of 1 h. Finally, dibutyltin dilaurate was added and stirred for additional 30 min. The reactant concentrations were adjusted to keep a constant NCO:OH molar ratio of 1:1 with a 5 wt% excess of H-MDI. The final concentration of PU in DMF was 0.2 g ml −1 . Polymer films were obtained by casting the solution onto silicone moulds and dried at 60 °C for 24 h. Supplementary Table S1 summarizes the amounts of chemicals used for the PU syntheses. Preparation of PU-based composites Composites reinforced with nano- and microplatelets were prepared following the procedure previously described by Libanori et al . [34] In summary, alumina platelets were first dispersed in a solution of PVP in DMF and kept under stirring for 12 h. Next, PU pellets (Elastollan) and a suspension of laponite in DMF (obtained through solvent exchange method) [34] , [35] were added to the alumina/PVP suspension. The resulting mixture was kept at room temperature and under stirring (600 r.p.m) until the polymer pellets were dissolved. The viscosity of the mixture was adjusted by removing DMF in an evaporator at 10 mbar and 60 °C (R-215 Rotavapor, Buchi, Switzerland) before casting the fluid on polyethylene plates using a doctor blade (height=1 mm). The remaining DMF was removed by placing the sample in a conventional oven (Memmert, UNE 200, Germany) at 60 °C for 24 h. The obtained composites were finally annealed at 130 °C for 3 h. Supplementary Table S2 depicts the composition of the platelet-reinforced composites investigated in this study. Preparation of patch–substrate composites Patch–substrate modules for mechanical and electrical testing were prepared by first assembling individual films (M0550, M1600, M3600 and M7000) into multilayered 0.4 × 5 cm 2 ribbons using the solvent-welding technique. For that purpose, a small amount of DMF was first applied on the two surfaces to be welded using a cotton swab. Pressure was manually applied onto the multilayer stack by squeezing the sample in between glass slides. The patch layers were assembled from the hardest to the softest material and subsequently welded onto a 5 cm × 5 cm × 0.19 mm M0040 substrate. The composition and thickness of each individual layer is indicated in Supplementary Table S3 . Finally, the samples were dried at 60 °C for 12 h in a vacuum oven. Two millimeter-wide dogbone samples were cut from the large M0040 substrate in the direction perpendicular to the multilayered ribbon to obtain patch–substrate modules with the architecture shown in Fig. 2a–c . For the resistance measurements, a 50 nm-thick gold layer was sputtered on the top of the stiffest layer ( Supplementary Fig. S7 ). Sputtering was carried out using a working distance of 50 mm, current of 40 mA and pressure of 2 × 10 −5 mbar for 200 s. Electrical contacts were made by gluing 100 μm-diameter copper wires to the gold layer using silver paste and an epoxy resin. Preparation of 3D heterogeneous composite The 3D heterogeneous composite shown in Fig. 1 f was prepared by first solvent welding 5 × 5 cm 2 individual layers of the compositions M0550, M1600, M3600, M7000, as described above. The resulting multilayered welded film was cut into 5 × 5 mm 2 patches using a scalpel. Finally, the patches were welded onto a 190 μm-thick M0040 substrate by applying DMF on both surfaces and manually pressing them together using glass slides. Patches welded on the top of the substrate were locally heated (60 °C) with a heating gun to ensure good adhesion between the materials and to remove the remaining solvent. Characterization For a detailed description of the experimental techniques used throughout this work, please refer to the Supplementary Methods . How to cite this article: Libanori, R. et al . Stretchable heterogeneous composites with extreme mechanical gradients. Nat. Commun. 3:1265 doi: 10.1038/ncomms2281 (2012).